Discovery of TaFeSb-based half-Heuslers with high thermoelectric performance 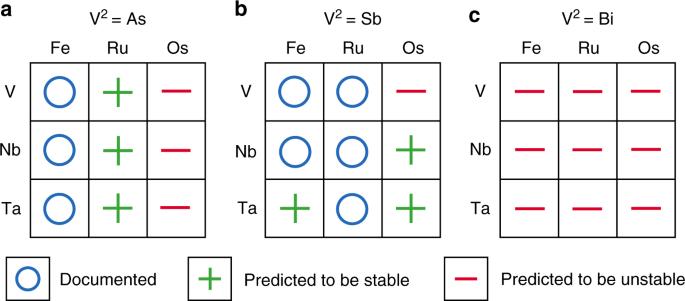Fig. 1 Thermodynamic stability calculation. Calculated stability of the V1-VIII-V2family (with V1= V, Nb, and Ta; VIII = Fe, Ru, and Os; and V2= As, Sb, and Bi) of half-Heusler compounds.aV1-VIII-As,bV1-VIII-Sb, andcV1-VIII-Bi Discovery of thermoelectric materials has long been realized by the Edisonian trial and error approach. However, recent progress in theoretical calculations, including the ability to predict structures of unknown phases along with their thermodynamic stability and functional properties, has enabled the so-called inverse design approach. Compared to the traditional materials discovery, the inverse design approach has the potential to substantially reduce the experimental efforts needed to identify promising compounds with target functionalities. By adopting this approach, here we have discovered several unreported half-Heusler compounds. Among them, the p-type TaFeSb-based half-Heusler demonstrates a record high ZT of ~1.52 at 973 K. Additionally, an ultrahigh average ZT of ~0.93 between 300 and 973 K is achieved. Such an extraordinary thermoelectric performance is further verified by the heat-to-electricity conversion efficiency measurement and a high efficiency of ~11.4% is obtained. Our work demonstrates that the TaFeSb-based half-Heuslers are highly promising for thermoelectric power generation. The ever-increasing energy consumption from fossil-fuel combustion has led to alarming environmental impacts. As one of the clean energy conversion techniques, thermoelectric power generation can harvest waste heat and convert it into electricity via the Seebeck effect [1] , [2] . However, the wide application of thermoelectric power generation systems requires significant improvements in the energy conversion efficiency, which essentially depends on the materials’ dimensionless figure-of-merit ( ZT ). It is defined as ZT = SσT /( κ lat + κ ele ), where S is the Seebeck coefficient, σ is the electrical conductivity, κ lat is the lattice thermal conductivity, κ ele is the electronic thermal conductivity, and T is the absolute temperature [3] , [4] , [5] , [6] , [7] . The transport parameters on which ZT depends are strongly interrelated with each other due to their different, and typically opposite, dependencies on carrier concentration and electronic structure [8] . Therefore, research on thermoelectric materials has focused on identifying approaches that can effectively decouple the key transport parameters for enhancing the ZT of existing materials [9] , [10] , [11] , [12] , [13] , [14] . In the meantime, relentless efforts have also been devoted to discovering promising new compounds that have unusual characteristics enabling favorable combinations of high electrical conductivity, large Seebeck coefficient, and low thermal conductivity. Historically, the materials discovery has mostly relied on the Edisonian trial and error approach. However, such a traditional process becomes increasingly time-consuming. As a result, there is a clear need for more efficient rational approaches to discovering new promising materials. This has provided the motivation for high-throughput methods and other theoretical approaches that use predictions of properties to identify candidate materials [15] , [16] . Yet a key challenge is to balance the reliability and cost in such studies. A consequence of the low reliability is that the predicted compounds (especially ones that have not yet been experimentally made) with promising thermoelectric performance may be experimentally identified as metastable or unstable. This is a particular challenge for thermoelectrics because a main approach for resolving the opposite dependencies of the transport properties, e.g., S and σ , is through unusual electronic structures, but unusual electronic properties are often found in calculations for unstable compounds, e.g ., due to unfavorable bonding. Thus, mere prediction of the thermoelectric properties for the missing compounds is not enough to guarantee experimental success. In fact, analysis of the thermodynamic stability for the unreported compounds and assessment of potential unknown competing phases could provide highly valuable guidance for the experimental efforts. It should be noted that careful experimental synthesis and evaluation of a compound are costly, while most theoretical calculations, especially as applied in high throughput modes, are relatively inexpensive. As such, it might be beneficial to use more sophisticated theoretical studies in predicting compounds before devoting the efforts for careful experimental study. Recently, Gautier et al. [17] investigated the thermodynamic stability of 400 unreported half-Heusler compounds and 54 of them were predicted to be stable. Subsequently, 15 compounds were successfully synthesized to verify their prediction. Similarly, Carrete et al. [18] performed the thermodynamic analysis for 450 half-Heusler compounds and predicted that 77 are stable. In addition, Zakutayev et al. [19] investigated the thermodynamic stability of the V-IX-IV family (V = V, Nb, and Ta; IX = Co, Rh, and Ir; and IV = C, Si, Ge, Sn, and Pb) of half-Heuslers. Their calculations indicated that among the 29 missing compounds, 8 are stable. TaCoSn, one of those predicted to be stable, was later successfully synthesized, confirming the prediction. Clearly, the inverse design approach [20] , which targets at the specific functionalities and involves with calculations of structure as well as thermodynamic stability and then followed by the experimental realization, is capable of significantly expediting the material discovery. In our work, we focused on the half-Heusler compounds, which are among the most promising candidates for thermoelectric applications. Thermodynamic stabilities of the V 1 -VIII-V 2 family (with V 1 = V, Nb, and Ta; VIII = Fe, Ru, and Os; and V 2 = As, Sb, and Bi) of half-Heuslers were systematically investigated. As a result, we have discovered 6 undocumented compounds and 5 of them are stable with the half-Heusler crystal structure. The p-type TaFeSb-based half-Heusler, one of the compounds discovered in this work, demonstrated a very promising thermoelectric performance. A peak ZT of~1.52 at 973 K and an average ZT of ~0.93 in the temperature range of 300~973 K were obtained. The high thermoelectric performance was further verified by the heat-to-electricity conversion efficiency measurement. A record high conversion efficiency of ~11.4% at the cold-side temperature of 317 K and hot-side temperature of 973 K was obtained. Thermodynamic stability analysis Systematic theoretical calculations on the V 1 -VIII-V 2 family (with V 1 = V, Nb, and Ta; VIII = Fe, Ru, and Os; and V 2 = As, Sb, and Bi) of half-Heusler phases were first conducted. In this family (27 compounds in total), 8 compounds have been documented to be stable while no experimental reports can be found for the remaining 19. Therefore, the crystal structure search for the missing compounds was conducted and the thermodynamic stability analysis of each compound with respect to all of the other competing phases was performed. The key aspect of the crystal structure search is that it allows us to check whether the half-Heusler structure is the true ground state rather than other possibly competing structures with the same 1:1:1 stoichiometry. We predict that 6 compounds (VRuAs, NbRuAs, TaRuAs, TaFeSb, NbOsSb, and TaOsSb) out of the missing 19 are stable, as shown in Fig. 1 . All of the predicted stable compounds are in the cubic structure ( F 43 m ), with the exception of NbRuAs that has an orthorhombic structure ( Pnma ). Some of these structures predicted agree quite well with the other theoretical calculations [18] , [21] . It should be noted that our prediction for NbRuAs differs from that of Carrete et al. [18] . We verified that the orthorhombic structure we found from the crystal structure prediction does have lower energy than the cubic structure they identified. The predicted energy difference is 25 meV per atom. In the following, we will focus mainly on TaFeSb, and the other five stable compounds will be reported elsewhere. Fig. 1 Thermodynamic stability calculation. Calculated stability of the V 1 -VIII-V 2 family (with V 1 = V, Nb, and Ta; VIII = Fe, Ru, and Os; and V 2 = As, Sb, and Bi) of half-Heusler compounds. a V 1 -VIII-As, b V 1 -VIII-Sb, and c V 1 -VIII-Bi Full size image For the thermodynamic stability of the V 1 -VIII-V 2 family, three criteria should be satisfied 
    Δμ _V^1 + Δμ _VIII + Δμ _V^2 = Δ H_f( V^1VIIIV^2);
 (1) 
    Δμ _i < 0,( i = V^1,VIII,V^2);
 (2) and 
    [ n_jΔμ _V^1 + m_jΔμ _VIII + q_jΔμ _V^2≤Δ H_f( V_n_j^1VIII_m_jV_q_j^2),;                                                          j = 1,...,t, ]
 (3) where \(\Delta \mu _i = \mu _i - \mu _i^0\) is the deviation of actual chemical potential of atomic species i during growth ( μ i ) from that of bulk elemental solid or gas phase ( \(\mu _i^0\) ), ∆ H f is the heat of formation, and \({\mathrm{V}}_{n_j}^1{\mathrm{VIII}}_{m_j}{\mathrm{V}}_{q_j}^2\) represents all of the known j competing phases, which provide a limitation to the broadening of the stable regions. Eq. ( 1 ) is for equilibrium growth, Eq. ( 2 ) is to prevent the precipitation of elemental phases of atomic species i , and Eq. ( 3 ) is to ensure that V 1 -VIII-V 2 half-Heuslers are stable against the formation of other competing phases. 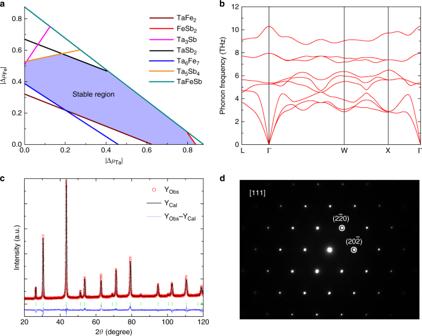Fig. 2 Theoretical prediction and experimental realization of TaFeSb half-Heusler.aPhase stability diagram for TaFeSb, where each line represents a known competing phase and the stable region is indicated in violet. It should be noted that\(\Delta \mu _{{\mathrm{Fe}}}\)and\(\Delta \mu _{{\mathrm{Ta}}}\)are both negative.b) Calculated phonon dispersion of TaFeSb.cRietveld refinement for the XRD pattern of the prepared TaFeSb in this work.dThe [111] zone-axis selected area electron diffraction pattern Figure 2a shows the two-dimensional phase stability diagram for TaFeSb with two independent quantities \(\Delta \mu _{{\mathrm{Fe}}}\) and \(\Delta \mu _{{\mathrm{Ta}}}\) . Six competing phases in the Ta-Fe-Sb system have been calculated to evaluate the stability of TaFeSb [22] , [23] . It should be noted that the Fe-Sb phase diagram includes a Fe 1.27 Sb phase. This phase is characterized by site disorder, and thus was not included in our calculations. A stable region for TaFeSb (marked by violet) exists with the consideration of all known potential competing phases. Such a large stability region for TaFeSb indicates that this compound should be synthesized experimentally. In addition, the lattice dynamical stability of TaFeSb was also examined and its phonon dispersion is shown in Fig. 2b . The absence of any imaginary phonon modes indicates the dynamical stability of the structure. To verify the theoretical prediction, we then carefully synthesized the TaFeSb compound by the ball-milling and hot-pressing method. Rietveld refinement for the XRD pattern of the prepared specimen indicates that the single-phase TaFeSb with half-Heusler structure was successfully synthesized. The obtained lattice parameter by Rietveld refinement is ~0.5938 nm (Fig. 2c ). The selected area electron diffraction (SAED) pattern for the prepared specimen viewed along the [111] direction is shown in Fig. 2d . The three-fold symmetry of the \(F\bar 43{\mathrm{m}}\) cubic structure along the [111] direction is well demonstrated by the SAED pattern and the corresponding atomic-resolution image (as shown in Supplementary Fig. 1 ). The lattice parameter (~0.59 nm) observed by STEM is consistent with the XRD results. Fig. 2 Theoretical prediction and experimental realization of TaFeSb half-Heusler. a Phase stability diagram for TaFeSb, where each line represents a known competing phase and the stable region is indicated in violet. It should be noted that \(\Delta \mu _{{\mathrm{Fe}}}\) and \(\Delta \mu _{{\mathrm{Ta}}}\) are both negative. b ) Calculated phonon dispersion of TaFeSb. c Rietveld refinement for the XRD pattern of the prepared TaFeSb in this work. d The [111] zone-axis selected area electron diffraction pattern Full size image Electronic properties of TaFeSb-based half-Heuslers Optimization of the thermoelectric performance of TaFeSb-based half-Heuslers was realized by tuning the carrier concentration via Ti-doping. In our work, Ta 1- x Ti x FeSb ( x = 0, 0.02, 0.04, 0.06, 0.08, 0.10, 0.12, 0.14, 0.16, and 0.18) samples were prepared by the ball-milling and hot-pressing method. All of the samples are highly dense with an average grain size of ~250 nm (as shown in Supplementary Fig. 2 ) and they are single-phase with high crystallinity (as shown in Supplementary Fig. 3 ). For simplicity, the thermoelectric properties of only some of the Ta 1- x Ti x FeSb specimens are shown in Fig. 3 , while the complete results can be found in Supplementary Fig. 4 . As shown in Fig. 3a , the electrical conductivity of the pristine TaFeSb is very low but it increases markedly with Ti-doping. Enhancement of the electrical conductivity should be attributed to the substantially increased hole concentration, as shown in Supplementary Fig. 5 . It is ~5.26 × 10 20 cm −3 for Ta 0.98 Ti 0.02 FeSb and ~2.03 × 10 21 cm −3 for Ta 0.84 Ti 0.16 FeSb. This indicates that Ti is a very efficient dopant for supplying a high concentration of holes to TaFeSb, which is similar to the case of Ti-doping in NbFeSb [24] , [25] . Due to the increased hole concentration, the Seebeck coefficient of Ta 1- x Ti x FeSb (with the exception of TaFeSb) is reduced gradually with increasing Ti concentration, as shown in Fig. 3b . It should be noted that the undoped TaFeSb is fully p-type over the whole temperature range and its Seebeck coefficient increases with temperature without showing any bipolar conduction despite its low hole concentration. This should be ascribed to the relatively large band gap of ~0.53 eV for TaFeSb, which is even larger than that of NbFeSb (~0.41 eV), as shown in Supplementary Fig. 6 . Optimization of the holeconcentration substantially improves the power factor of TaFeSb-based half-Heuslers, as shown in Fig. 3c . The room-temperature power factor is ~45 μW cm −1 K −2 for Ta 0.84 Ti 0.16 FeSb and its peak power factor can be as large as ~56 μW cm −1 K −2 , thus leading to its high average power factor of ~52 μW cm −1 K −2 in the temperature range between 300 and 973 K. Such a high power factor outperforms most of the other state-of-the-art half-Heusler compounds, e.g., (Ti/Zr/Hf)CoSb [26] , [27] , [28] , (Ti/Zr/Hf)NiSn [29] , [30] , [31] , [32] , [33] , ZrNiPb [34] , and NbCoSn [35] , [36] . The origin of the high electronic thermoelectric performance of TaFeSb-based half-Heuslers can be partially ascribed to the unique electronic band structure, as shown in Fig. 3d . The valence band maximum locates at the L-point (with a carrier pocket degeneracy of four), where two valence bands (with an orbital degeneracy of two) effectively converge and thus leading to a very high valley degeneracy ( N v ) of eight (as shown in Supplementary Fig. 7 ). The thermoelectric figure of merit ZT is closely correlated with the materials’ parameter B , where \(B \propto N_{\mathrm{V}}\mu \left( {m^ \ast } \right)^{3/2}/\kappa _{{\mathrm{lat}}}\) ( μ is the mobility and m * is the effective mass) [1] , [37] . Therefore, the high band degeneracy of TaFeSb is highly beneficial for realizing the large power factor. Fig. 3 Electronic properties of TaFeSb-based half-Heuslers. Temperature-dependent a electrical conductivity, b Seebeck coefficient, and c power factor of Ta 1- x Ti x FeSb ( x = 0, 0.02, 0.04, 0.06, 0.08, 0.12, and 0.16). d Band structure of TaFeSb Full size image Thermal conductivities of TaFeSb-based half-Heuslers Comparison of the thermal conductivity between the undoped NbFeSb and TaFeSb is shown in Supplementary Fig. 8 . The room-temperature thermal conductivity is ~14 W m −1 K −1 for NbFeSb and it is only ~8.8 W m −1 K −1 for TaFeSb. To understand the difference in lattice thermal conductivity, phonon dispersion relations for NbFeSb and TaFeSb were calculated as shown in Supplementary Fig. 9 . TaFeSb has overall lower phonon frequencies than those of NbFeSb. The acoustic phonon velocity is lower in TaFeSb compared to NbFeSb. Usually, the phonon velocity can simply be approximated by the low frequency sound velocity [38] . The measured sound velocity is 2907 m s −1 for TaFeSb but is 3473 m s −1 for NbFeSb (as shown in Supplementary Fig. 10 ). According to the kinetic theory, the lattice thermal conductivity can be expressed as \(\kappa _{{\mathrm{lat}}}{\mathrm{ = }}\frac{1}{3}C_{\mathrm{v}}v_{{\mathrm{ph}}}l\) , where C v is the heat capacity per unit volume, v ph is the phonon velocity, and l is the phonon mean free path [39] . Therefore, the lower phonon velocity of TaFeSb can account for its lower thermal conductivity compared to NbFeSb. Although the electrical conductivity of TaFeSb has been substantially increased by Ti-doping (which effectively increases the electronic thermal conductivity via the Wiedemann-Franz law κ ele = LσT , where L is the Lorenz constant), the total thermal conductivity of Ta 1- x Ti x FeSb demonstrates a noticeable reduction with increasing Ti concentration (as shown in Fig. 4a ). The composition-dependent lattice thermal conductivity of Ta 1- x Ti x FeSb is calculated and shown in Fig. 4b . It demonstrates a monotonic reduction with respect to Ti concentration. The room-temperature lattice thermal conductivity is ~8.8 W m −1 K −1 for TaFeSb but is only ~3.1 W m −1 K −1 for Ta 0.84 Ti 0.16 FeSb, a reduction of ~65%. Such a significant phonon scattering should be ascribed mainly to the presence of point defects induced by Ti-doping at the Ta site. The substantial difference in atomic mass between Ti (~47.87) and Ta (~180.95) leads to the strong scattering that effectively disrupts the phonon propagation. 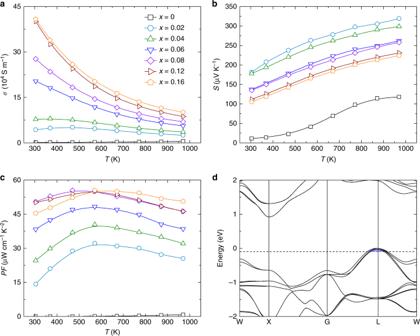Fig. 3 Electronic properties of TaFeSb-based half-Heuslers. Temperature-dependentaelectrical conductivity,bSeebeck coefficient, andcpower factor of Ta1-xTixFeSb (x= 0, 0.02, 0.04, 0.06, 0.08, 0.12, and 0.16).dBand structure of TaFeSb By alloying the Ta 0.84 Ti 0.16 FeSb composition with VFeSb, the lattice thermal conductivity can be further reduced, as shown in Fig. 4c and Supplementary Fig. 11e . The room-temperature lattice thermal conductivity is ~3.1 W m −1 K −1 for Ta 0.84 Ti 0.16 FeSb and is only ~2.3 W m −1 K −1 for Ta 0.74 V 0.1 Ti 0.16 FeSb, a decrease of ~26%. Fig. 4 Thermal conductivity of TaFeSb-based half-Heuslers. a Temperature-dependent thermal conductivity of Ta 1- x Ti x FeSb, b composition-dependent room-temperature lattice thermal conductivity of Ta 1- x Ti x FeSb, and c comparison of lattice thermal conductivity between Ta 0.84 Ti 0.16 FeSb and Ta 0.74 V 0.1 Ti 0.16 FeSb Full size image ZT and energy conversion efficiency of TaFeSb-based half-Heuslers Benefitting from the simultaneous enhancement in power factor and reduction in thermal conductivity, the thermoelectric figure of merit of TaFeSb-based half-Heuslers can be effectively improved after Ti-doping. The thermoelectric performance of Ta 1- x Ti x FeSb increases with the Ti concentration and Ta 0.84 Ti 0.16 FeSb achieves a high peak ZT of ~1.39 at 973 K (as shown in Fig. 5a ). As mentioned earlier, by alloying Ta 0.84 Ti 0.16 FeSb with VFeSb, it is possible to further reduce the thermal conductivity and the power factor remains similar when V concentration is less than 15 at.% (as shown in Supplementary Fig. 11c ). Therefore, the thermoelectric performance of TaFeSb-based half-Heuslers can be further improved and Ta 0.74 V 0.1 Ti 0.16 FeSb achieves a peak ZT of ~1.52 at 973 K. To demonstrate the repeatability of our results, Ta 0.74 V 0.1 Ti 0.16 FeSb has been prepared in five different batches and the thermoelectric properties are quite similar (as shown in Supplementary Fig. 12 ). The thermal stability of Ta 0.74 V 0.1 Ti 0.16 FeSb was further characterized by repeatedly measuring the same specimen five times and the thermoelectric properties are also comparable (as shown in Supplementary Fig. 13 ). This indicates that the high thermoelectric performance of Ta 0.74 V 0.1 Ti 0.16 FeSb is very stable and repeatable. Comparison of the thermoelectric performance between the TaFeSb-based half-Heuslers with the other p-type state-of-the-art half-Heusler compounds [24] , [25] , [26] , [27] is shown in Fig. 5b . Clearly, Ta 0.74 V 0.1 Ti 0.16 FeSb outperforms all of the other half-Heuslers over the whole temperature range between 300 and 973 K. The average ZT is further calculated by the integration method (with a fourth-order polynomial for fitting the ZT curve) between 300 and 973 K and comparison of the average ZT is shown in Fig. 5c . The average ZT s are ~0.53 for Hf 0.8 Ti 0.2 CoSb 0.8 Sn 0.2 [26] , ~0.57 for Nb 0.8 Ti 0.2 FeSb [25] , ~0.67 for Nb 0.88 Hf 0.12 FeSb [24] , and ~0.81 for ZrCoBi 0.65 Sb 0.15 Sn 0.2 [40] , all of which are lower than ~0.82 for Ta 0.84 Ti 0.16 FeSb and ~0.93 for Ta 0.74 V 0.1 Ti 0.16 FeSb. The high thermoelectric performance of Ta 0.74 V 0.1 Ti 0.16 FeSb was further verified by the heat-to-electricity conversion efficiency measurement. As shown in Fig. 5d , the measured peak efficiency of Ta 0.74 V 0.1 Ti 0.16 FeSb can be as large as ~11.4% at the cold-side temperature of 317 K and hot-side temperature of 973 K. This is a record high efficiency for a single leg based on half-Heusler thermoelectric materials. Our results demonstrate that the TaFeSb-based half-Heuslers are quite promising for thermoelectric power generation. Fig. 5 Dimensionless thermoelectric figure of merit of TaFeSb-based half-Heuslers. a Temperature-dependent ZT of Ta 1- x Ti x FeSb, b comparison of the ZT between Ta 0.74 V 0.1 Ti 0.16 FeSb and the other state-of-the-art p-type half-Heuslers [24] , [25] , [26] , [27] , c comparison of the average ZT (in the range between 300 and 973 K) between TaFeSb-based half-Heuslers and the other state-of-the-art p-type half-Heuslers, and d the measured hot-side temperature-dependent heat-to-electricity conversion efficiency of Ta 0.74 V 0.1 Ti 0.16 FeSb as compared with state-of-the-art p-type half-Heuslers ZrCoBi 0.65 Sb 0.15 Sn 0.2 [40] and Nb 0.8 Ti 0.2 FeSb [25] . The cold-side temperature is fixed at 300 K for the calculation of efficiency (solid line) Full size image In summary, thermodynamic stability analysis was performed for the V 1 -VIII-V 2 family (with V 1 = V, Nb, and Ta; VIII = Fe, Ru, and Os; and V 2 = As, Sb, and Bi) of half-Heuslers. We predicted that six compounds (VRuAs, NbRuAs, TaRuAs, TaFeSb, NbOsSb, and TaOsSb) in this family should be stable. To verify this prediction, the TaFeSb-based half-Heuslers were synthesized and their thermoelectric performance was optimized. Our results indicated that Ta 0.74 V 0.1 Ti 0.16 FeSb can achieve a peak ZT of ~1.52 at 973 K, outperforming all of the other state-of-the-art p-type half-Heusler materials. More importantly, the heat-to-electricity conversion efficiency was also measured for the TaFeSb-based half-Heuslers and the maximum efficiency can be as large as ~11.4% at the cold-side temperature of 317 K and hot-side temperature of 973 K. Our work demonstrated that the TaFeSb-based half-Heuslers are quite promising for thermoelectric power generation. Synthesis TaFeSb-based half-Heuslers were prepared by a two-step ball-milling and hot-pressing method. In the first step, Ta turnings (99.98%; Atlantic Metals & Alloys) and Sb ingots (99.999%; Alfa Aesar) were loaded into a stainless-steel jar under an argon atmosphere in a glove box and ball-milled for 15 h. Afterward, Fe granules (99.8%; Alfa Aesar), Ti granules (99.99%; Alfa Aesar), and V pieces (99.7%; Alfa Aesar) were added for another 20 h ball milling. The ball-milling process was conducted using a SPEX 8000 M Mixer/Mill. The ball-milled powders were compacted to a disk by a direct-current-induced hot-pressing at about 1123 K for 2 min and under the pressure of ~80 MPa. Thermoelectric properties measurement The Seebeck coefficient and electrical conductivity were simultaneously obtained by a commercial (ZEM-3, ULVAC) system in helium atmosphere. The thermal conductivity κ = DC p ρ was calculated from the thermal diffusivity D (LFA 457, Netzsch), specific heat C p (DSC 404 C; Netzsch), and mass density ρ (Archimedes’ kit). Hall carrier concentrations ( n H ) were measured using a commercial system (PPMS Dynacool, Quantum Design) with a magnetic field of ±3 T and an electrical current of 8 mA. Efficiency measurement The thermoelectric material (referenced as leg in the following discussion) was polished to the size of 2.6 × 2.7 mm 2 in cross-section and ~11 mm in length. The cold-side temperature was maintained at around 287–317 K by water circulation. The experiments were conducted under high vacuum (below 10 −6 mbar) to reduce the parasitic conduction and convection losses. To measure conversion efficiency ( η ), the input power from the hot side ( Q in ) and the generated power ( P ) from the thermoelectric leg were measured at the same time. The direct measurement of Q in is a greatly challenging due to the heavy heat loss at high temperature. According to Fourier’s law, a bulk polycrystalline graphite with measured geometry and thermal conductivity was placed below the cold-side to measure the heat flow out of the cold-side ( Q out ). The thermal conductivity of the bulk polycrystalline graphite was confirmed by the method described above in the discussion on thermoelectric properties measurement. In order to measure temperature differences of the leg and graphite bulk, K-type thermocouples were embedded at the interfaces. It should be noted that the hot-side temperature of graphite can be regarded as the cold-side temperature of the leg if the setup is working under a large pressure. The total Q in equals the sum of Q out , P , and radiation loss from the leg ( Q rad ). Therefore, the conversion efficiency ( η ) can be written as the following 
    η = P/Q_in = P/Q_out + P + Q_rad. (4) Since Q rad cannot be directly measured, in real measurement Q in is composed of Q out and P , which leads to the measurement error of η . By tuning the current in the circuit, a series of Q in , P can be measured at the same time. Therefore, both maximum η and P can be found. The estimated radiation loss based on the finite difference method is about 1–6% of the total heat flow in. For p -type thermoelectrics, the measured open circuit voltage should be smaller since the Seebeck coefficient of copper is a positive number, which can be given by a following empirical function [41] 
    [ S_Cu( T ) = 0.041T[ exp(  - T/93) + 0.123 - 0.442/1 + (T/172.4)^3]+ 0.804,;                                                           70K < T < 1000K. ] (5) The Seebeck coefficient of copper is ~6 μV K −1 at 973 K, and the measured output power at 973 K is underestimated by about 5-6%. Microstructural characterization Phase identification was carried out by X-ray diffraction (XRD) on a PANalytical multipurpose diffractometer with an X’Celerator detector (PANalytical X’Pert Pro). 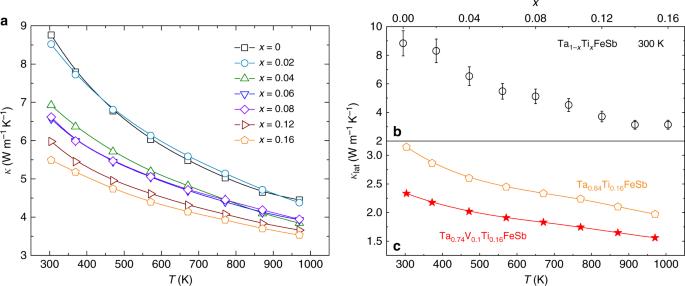Fig. 4 Thermal conductivity of TaFeSb-based half-Heuslers.aTemperature-dependent thermal conductivity of Ta1-xTixFeSb,bcomposition-dependent room-temperature lattice thermal conductivity of Ta1-xTixFeSb, andccomparison of lattice thermal conductivity between Ta0.84Ti0.16FeSb and Ta0.74V0.1Ti0.16FeSb 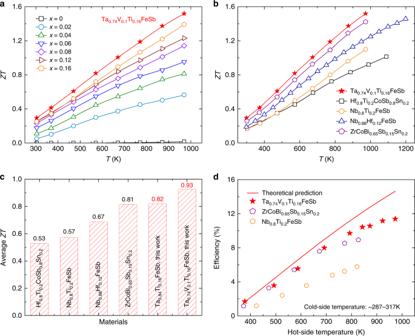Fig. 5 Dimensionless thermoelectric figure of merit of TaFeSb-based half-Heuslers.aTemperature-dependentZTof Ta1-xTixFeSb,bcomparison of theZTbetween Ta0.74V0.1Ti0.16FeSb and the other state-of-the-art p-type half-Heuslers24,25,26,27,ccomparison of the averageZT(in the range between 300 and 973 K) between TaFeSb-based half-Heuslers and the other state-of-the-art p-type half-Heuslers, anddthe measured hot-side temperature-dependent heat-to-electricity conversion efficiency of Ta0.74V0.1Ti0.16FeSb as compared with state-of-the-art p-type half-Heuslers ZrCoBi0.65Sb0.15Sn0.240and Nb0.8Ti0.2FeSb25. The cold-side temperature is fixed at 300 K for the calculation of efficiency (solid line) The morphology and microstructures were characterized by a field emission scanning electron microscope (FESEM, LEO 1525). Selected area electron diffraction pattern and HAADF-STEM images were obtained by a JEM-ARM 200F TEM operated at 200 kV. Bandgap measurement Fourier transform infrared spectroscopy (FTIR) was performed to derive the optical band gap based on the Kramers-Kronig analysis of the reflectance. The FTIR was conducted using a Nicolet iS50 FT-IR spectrometer with a Spectra-Tech model 500 series variable angle specular reflectance accessory at room temperature. Sound velocity measurement Sound velocity measurements were carried out using a RITEC Advanced Ultrasonic Measurement System RAM-5000. The system realizes the pulse-echo method of time propagation measurements with an accuracy of about 10 −3 µs. To generate longitudinal (L) and shear (S) ultrasonic bulk waves, Olympus transducers V129-RM (10 MHz) and V157-RM (5 MHz) were used. Propylene glycol and SWC (both from Olympus) were used as couplant materials for the L and S modes, respectively. Thickness measurements were carried out using a Mitutoyo ID-HO530 device. All data were obtained at 300 K. Theoretical calculations We searched for stable V 1 -VIII-V 2 half-Heusler crystal structures up to 18 atoms per unit cell using the global optimization particle swarm method as implemented in the CALYPSO code [42] , [43] . At least 2000 structures were calculated during each search. The key feature of the CALYPSO method is the ability to rapidly identify ground-state structures with knowledge only of the chemical composition. Details of the algorithm and applications have been discussed elsewhere [44] , [45] , [46] . The first-principles calculations of the formation energy were performed using the projector-augmented wave (PAW) method as implemented in the VASP code [47] , [48] . The electronic structures were obtained with the general potential linearized augmented plane wave (LAPW) method as implemented in the WIEN2k code [49] . This enabled us to realize structure optimization and hybrid functional calculations using VASP, which is time consuming and has the potential compatibility issue (with CALYPSO) in WIEN2K, as well as allowing the convenience of the later transport calculations using WIEN2K. The Perdew, Burke, and Ernzerhof (PBE-GGA) type functional was used for the structural optimization within VASP [50] . Because of the sensitivity of thermodynamic stability, the 3 p 6 3 d 3 4 s 2 (V), 4 p 6 4 d 4 5 s 1 (Nb), 5 p 6 5 d 3 6 s 2 (Ta), 3 p 6 3 d 6 4 s 2 (Fe), 4 p 6 4 d 7 5 s 1 (Ru), 5 p 6 5 d 6 6 s 2 (Os), 4 s 2 4 p 3 (As), 5 s 2 5 p 3 (Sb), and 5 d 10 6 s 2 6 p 3 (Bi) states were treated as valence electrons of PAW pseudopotentials. These were used with kinetic energy cutoffs of 520 eV. We conducted tests to ensure that this was adequate. The k-point meshes for sampling the Brillouin zone were at a grid spacing of 2 π × 0.032 Å or better, including the hybrid functional calculations. Harmonic phonons were obtained with real space supercells using the PHONOPY code [51] . Band structure and density of states (DOS) calculations were conducted by using the modified Becke–Johnson (mBJ) potential of Tran and Blaha [52] , [53] . This mBJ potential gives band gaps in agreement with experiment for a wide variety of simple semiconductors and insulators [54] , [55] . In the present case, our calculated band gap of 0.9 eV is larger than the experimental value, perhaps due to site disorder in the half-Heusler structure. We also cross-checked the band gaps using the hybrid Heyd–Scuseria–Ernzerhof (HSE06) functional [56] , which also supports a larger band gap. Spin–orbit coupling (SOC) was included in electronic structure calculations, as the spin–orbit splitting may be very large for heavy elements. We used LAPW sphere radii of 2.5 bohr for TaFeSb. A basis set cutoff, K max , determined by the criterion R min K max = 9.0, was used. Here, R min denotes the minimum atomic radius of elements.